Thermally robust and porous noncovalent organic framework with high affinity for fluorocarbons and CFCs Metal-organic and covalent organic frameworks are porous materials characterized by outstanding thermal stability, high porosities and modular synthesis. Their repeating structures offer a great degree of control over pore sizes, dimensions and surface properties. Similarly precise engineering at the nanoscale is difficult to achieve with discrete molecules, since they rarely crystallize as porous structures. Here we report a small organic molecule that organizes into a noncovalent organic framework with large empty pores. This structure is held together by a combination of [N–H···N] hydrogen bonds between the terminal pyrazole rings and [π···π] stacking between the electron-rich pyrazoles and electron-poor tetrafluorobenzenes. Such a synergistic arrangement makes this structure stable to at least 250 °C and porous, with an accessible surface area of 1,159 m 2 g −1 . Crystals of this framework adsorb hydrocarbons, CFCs and fluorocarbons—the latter two being ozone-depleting substances and potent greenhouse species—with weight capacities of up to 75%. Chemistry of porous materials has been revolutionized with the development of crystallographically ordered hybrid structures known as metal-organic (MOFs) [1] and covalent organic (COFs) [2] , [3] frameworks. These materials are characterized by high thermal stability, exceptional surface areas and highly modular syntheses, which allow facile modification of pore sizes, shapes and polarities. While this strategy allows superior control over pore properties, it comes with a price. As extended crystalline materials, MOFs and COFs are essentially impossible to dissolve without decomposition, and thus the scope of their solution-phase characterization and processability is limited. Significant advances have been made in the ability to deposit MOFs and COFs on surfaces [4] , [5] , [6] , but considerable benefits could still come from robust porous structures constructed from discrete small molecules. Unfortunately, highly porous crystal structures of discrete molecules are rare and difficult to predict a priori [7] ; furthermore, even when a small molecule can be organized into a porous structure, such structures are typically fragile after solvent removal. Recent work by Chen [8] , [9] , Cooper [10] , [11] , [12] , Mastalerz [13] , [14] , [15] , [16] , [17] , [18] , [19] and others [20] , [21] , [22] , has resulted in molecular crystals characterized by high porosity. These noncovalently held structures can be intrinsically or extrinsically porous. The former are based on macrocycles or molecular capsules that contain a large central void; organization of these within the crystal results in an extended structure that replicates individual molecules’ porosities. In the latter case, the molecule itself is inherently nonporous, and all porosity comes as the consequence of crystal packing. Mastalerz et al. have reported intrinsically porous molecular crystals with surface areas over 3,500 m 2 g −1 (ref. 18 ), and extrinsically porous ones with surface areas >3,000 m 2 g −1 (ref. 14 ). However, some of these highly porous structures are based on hydrolytically fragile imines and boronate esters [4] , [23] . Here we present the synthesis and characterization of a trispyrazole 1 that organizes into a robust, extrinsically porous noncovalent organic framework (nCOF) through a combination of [π···π] stacking [24] and hydrogen bonding [25] , [26] . Crystals of 1 capture as much as 75% of their weight in hydrocarbons and fluorocarbons, which is relevant to both fuel processing and capture of greenhouse species. Synthesis of trispyrazole 1 The synthesis of 1 ( Fig. 1 ) commenced with the commercially available 4-iodopyrazole ( 2 ). The masking of its N–H bond with a trityl (Ph 3 C–) group gave compound 3 , which was subjected to a palladium-catalysed coupling with an excess of 1,2,4,5-tetrafluorobenzene to produce intermediate 4 . In 4 , only one of the two C–H bonds of tetrafluorobenzene was replaced with a functionalized pyrazole moiety. Another palladium-catalysed coupling followed, combining 3.3 equivalents of 4 with 1,3,5-triiodobenzene and resulting in the trigonal precursor 5 . The trityl groups in 5 were removed by acidic treatment, and subsequently replaced with the tert -butyloxycarbonyl (Boc) group. Heating of a solution of 6 in N , N -dimethylformamide (DMF) and MeOH for 1 day at 80 °C resulted in single crystals of compound 1 ; crystals are formed before the solution is cooled to room temperature. This procedure utilized previously reported protocols for the in situ deprotection of Boc group [27] and concurrent binding to metals [28] , [29] . 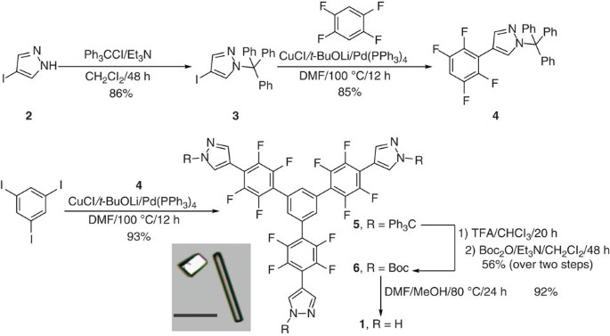Figure 1: Synthesis of compound 1. Reaction of 4-iodopyrazole2with trityl chloride produces protected pyrazole3, which is then coupled to 1,2,4,5-tetrafluorobenzene to give4. Threefold coupling of4with 1,3,5-triiodobenzene generates trigonal precursor5. Series of protecting group manipulations produces1. Ph, phenyl; Et, ethyl; Me, methyl; DMF,N,N-dimethylformamide; TFA, trifluoroacetic acid;t-Bu,tert-butyl; Boc,tert-butyloxycarbonyl. Inset shows an image of typical crystals of1. Scale bar, 200 μm. Figure 1: Synthesis of compound 1. Reaction of 4-iodopyrazole 2 with trityl chloride produces protected pyrazole 3 , which is then coupled to 1,2,4,5-tetrafluorobenzene to give 4 . Threefold coupling of 4 with 1,3,5-triiodobenzene generates trigonal precursor 5 . Series of protecting group manipulations produces 1 . Ph, phenyl; Et, ethyl; Me, methyl; DMF, N , N -dimethylformamide; TFA, trifluoroacetic acid; t -Bu, tert -butyl; Boc, tert -butyloxycarbonyl. Inset shows an image of typical crystals of 1 . Scale bar, 200 μm. Full size image Crystallographic analysis of compound 1 Single-crystal X-ray diffraction data on 1 were obtained with the use of synchrotron radiation (see Supplementary Data 1 for the crystallographic information file—CIF, and Supplementary Methods for the discussion of data collection and refinement). The asymmetric unit contains parts of two crystallographically distinct molecules, one of which has a C 2 axis dissecting it. Several aspects of this structure are shown in Fig. 2 . The three arms of 1 twist in a propeller-like fashion out of the plane of the central ring, forming angles of 33.7°, 33.8° and 46.3° (in the more symmetric molecule of 1 , all three angles are 32.8°). Each molecule of 1 establishes short contacts with 12 of its neighbours: six [N–H···N] hydrogen bonds, which create a hexagonal two-dimensional lattice, and six [π···π] stacking arrangements, which propagate these layers into the third dimension. Pyrazoles at the end of each arm of 1 establish hydrogen bonds with two adjacent molecules ( Fig. 2a ) [30] , [31] . These bonds are close to each other in length: N···H distances vary between 1.81 and 1.91 Å (lengths of N–H bonds involved in hydrogen bonding have been normalized to values obtained from neutron diffraction, see ref. 32 ), while N···N distances vary between 2.78(1) and 2.854(9) Å. Control of inter-layer relationships is achieved through [π···π] stacking of the electron-poor tetrafluorinated aromatic rings with the relatively electron-rich pyrazoles ( Fig. 2b ), but this relationship is highly unsymmetric. In each molecule of 1 , the most deplanarized of the three arms engages in the predicted [π···π] stacking with its ‘top’ and ‘bottom’ neighbours. These AB stacks are symmetric, with centroid–centroid distances between the pyrazole and tetrafluorobenzene rings being 3.68 Å and 3.69 Å (centroid–centroid distances are quoted because ring planes are not parallel and thus interplanar distance cannot be determined, vide infra). The angles between the adjacent planes of pyrazole and tetrafluorobenzene rings is 11.2° and 9.7°. A more peculiar situation is observed with the other two ‘arms’ of compound 1 . In these, the top and the bottom neighbours are no longer equivalent. One establishes a pair of [π···π] stacking interactions characterized by centroid–centroid distances of 3.42 and 3.50 Å and interplanar angles of 10.3 and 11.4°, respectively. But the other neighbour establishes an oddly slipped [π···π] stacking, in which centroids of tetrafluorobenzene and pyrazole rings reside quite far from each other at 5.28 Å. In fact, the closest two rings are two tetrafluorobenzenes, with a centroid–centroid distance of 4.08 Å, and essentially parallel arrangement of the planes (interplanar angle of 0.49°). This arrangement—which is repeated in the third arm of 1 —is caused by the steric mismatch of the central benzene ring with the ‘pyrazole triad’ that resides above it in the next layer, and so one arm of the molecule must sacrifice favourable [π···π] stacking interactions to accommodate this dimensional difference. 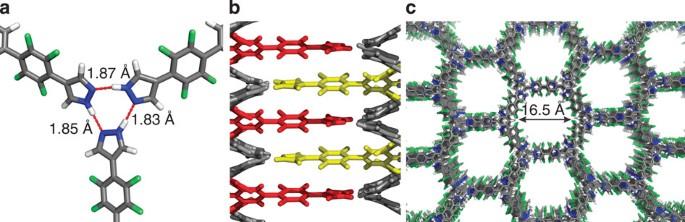Figure 2: Crystal structure of compound 1. Three pyrazoles come together in each of the layers (a) forming a triplet of hydrogen bonds. Each pyrazole engages in [π···π] stacking interactions with six of its neighbours, wherein electron-rich pyrazoles stack with electron-poor tetrafluorobenzene rings (b). Overall, a hexagonal network results, with infinite fluorine-lined channels protruding throughout the structure along the crystallographiccaxis (c). Figure 2: Crystal structure of compound 1. Three pyrazoles come together in each of the layers ( a ) forming a triplet of hydrogen bonds. Each pyrazole engages in [π···π] stacking interactions with six of its neighbours, wherein electron-rich pyrazoles stack with electron-poor tetrafluorobenzene rings ( b ). Overall, a hexagonal network results, with infinite fluorine-lined channels protruding throughout the structure along the crystallographic c axis ( c ). Full size image Overall, a three-dimensional network results, with infinite one-dimensional channels protruding throughout the crystal along the crystallographic c axis; these channels are lined with fluorines and have a diameter of ~16.5 Å ( Fig. 2c ). Layers of this crystal structure can be described as having hnb topology [33] with two distinct kinds of vertices, edges and faces; adjacent layers are offset so that two faces of different kinds stack with each other. All structural elements of 1 are essential in producing the infinite porous structure: pyrazole is needed to establish the hydrogen-bonding pattern within the two-dimensional layers, while the electron-poor perfluorinated ring can favourably [π···π] stack with the relatively electron-rich pyrazole. Characterization of stability Compound 1 is colourless and remarkably stable to solvents, acids and bases. Visual inspection of the crystals shows no signs of crystal decomposition or dissolution in off-the-shelf dichloromethane, hexanes, toluene or acetone for at least 30 days. Furthermore, after crystals of 1 treated with these solvents were dried and subjected to powder X-ray diffraction (PXRD) analysis, their PXRD patterns were virtually identical to those of the original samples ( Supplementary Fig. 1 ). Similar analysis confirmed the material to be stable to deionized water at 25 °C for at least 30 days, and at 100 °C for at least 7 days. Compound 1 > also tolerated acids (1 M HCl) and bases (2 M NaOH) at 25 °C for at least 30 days. It is sparingly soluble in dimethyl sulfoxide (DMSO) at 25 °C, but its solubility in this solvent considerably increases with temperature. While many organic molecules form crystal structures with large apparent empty spaces, those spaces are typically occupied by solvent molecules, and tend to collapse upon solvent removal [15] . Compound 1 is different in that respect. Its single-crystal X-ray structure—refined from the data collected at −173°C—revealed significant electron density within the pores attributed to disordered solvent. However, all of that solvent appears to leave the pores within minutes at 25 °C without any observable loss of crystallinity. Thermogravimetric analysis (TGA, Fig. 3a ) of 1 was performed in both air (red trace in Fig. 3a ) and nitrogen (blue trace), confirming the absence of solvent in the as-synthesized crystal. After air-drying, heating of this material does not result in any weight loss up until 360 °C, significantly above the boiling points of all the solvents used in the synthesis. We speculate that the perfluorinated material associates only very weakly with the hydrophilic solvents—DMF, MeOH and residual H 2 O—used in its synthesis. At 360 °C, compound 1 loses ~11% of its weight under both nitrogen and air. Oddly, the material recovered from the TGA experiment that was heated slightly above 360 °C shows almost exactly the same elemental analysis (within 3% for all elements) as the pristine nCOF. This observation could suggest partial sublimation, but it is unclear why this should result in a relatively sharp 11% weight loss observed. Isolation of minor amounts of the sublimed products from the TGA vent tubing and their characterization by nuclear magnetic resonance (NMR) suggested a complex mixture of products. Overall, TGA of 1 is complicated by its relatively low sublimation point (versus MOFs and COFs), and multiple apparent decomposition pathways. Slightly above 400 °C, the second stage of weight-loss begins; in a nitrogen-based TGA experiment, about 50% of the original weight remains even at 900 °C, while in air the entire sample is consumed below 600 °C. 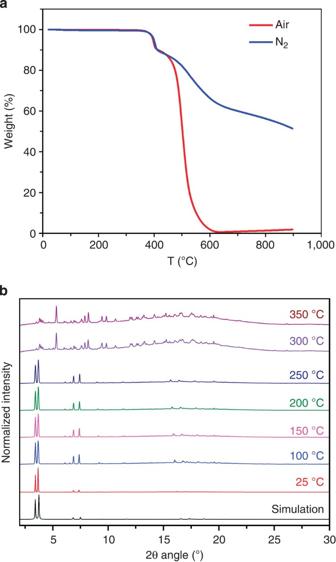Figure 3: Thermal stability of compound 1. (a) Thermogravimetric analysis (TGA) in nitrogen (blue trace) and air (red trace) shows no weight loss until 360 °C, suggesting that no solvent was included in the crystal structure of1. Between 360 and 400 °C, compound1loses ~11% of its weight regardless of the carrier gas. Beyond 400 °C, slow decomposition of the material ensues under nitrogen, and much faster one under air. (b) Variable temperature powder X-ray diffraction (PXRD) revealed no change in structure until at least 250 °C. Beyond that temperature, an irreversible phase change occurs. Structure of this new crystalline phase was not determined. Figure 3: Thermal stability of compound 1. ( a ) Thermogravimetric analysis (TGA) in nitrogen (blue trace) and air (red trace) shows no weight loss until 360 °C, suggesting that no solvent was included in the crystal structure of 1 . Between 360 and 400 °C, compound 1 loses ~11% of its weight regardless of the carrier gas. Beyond 400 °C, slow decomposition of the material ensues under nitrogen, and much faster one under air. ( b ) Variable temperature powder X-ray diffraction (PXRD) revealed no change in structure until at least 250 °C. Beyond that temperature, an irreversible phase change occurs. Structure of this new crystalline phase was not determined. Full size image To probe the structural changes that occur with heating, we also performed variable-temperature PXRD study of 1 ; results, shown in Fig. 3b , suggest that the crystal phase does not change until at least 250 °C. Small changes in unit cell parameters are observed with increasing temperature, but those are under 4% of individual unit cell dimensions (see Supplementary Figs 2 and 3 ) and are thus not suggestive of a phase change. At higher temperatures, the PXRD pattern changes markedly and irreversibly, but the material still appears largely crystalline, although the broad peak in PXRD pattern baseline may suggest a contribution from an amorphous phase. Differential scanning calorimetry (DSC) measurements show a sharp peak at 285 °C, consistent with a phase change (see Supplementary Fig. 4 ). The discrepancy between the apparent decomposition temperatures obtained from TGA and PXRD measurements could be rationalized by the possibility that the phase change observed by PXRD is not associated with weight loss. Compound 1 can be sublimed in high vacuum (0.03 mm Hg) at 250 °C during the course of 48 h. The obtained material is crystalline, but its PXRD pattern ( Supplementary Fig. 5 ) matches neither the one of the as-synthesized sample of 1 , nor the one observed after 1 was heated to >300 °C; this new phase is also completely nonporous. This finding, along with the irreversible thermal phase change observed by variable temperature PXRD ( Fig. 3b ), suggests that the porous structure of 1 is a kinetic rather than a thermodynamic product. Guest sorption within the pores of 1 Gas sorption within the pores of 1 was probed using nitrogen, oxygen and CO 2 as guests. On the basis of the nitrogen adsorption isotherm ( Fig. 4 ), the Brunauer–Emmett–Teller surface area of 1 was determined to be 1,159 m 2 g −1 , and the pore volume was estimated at 51%. These values agree reasonably well with those calculated from crystal structure data using CrystalExplorer and PLATON [34] software packages: 1,481 m 2 g −1 and 56%, respectively [35] . Using non-linear density functional theory (NLDFT) calculations, pores were estimated to be ~11 Å in diameter ( Supplementary Fig. 6 ); this result is significantly lower than that measured from the crystal structure, but existing models may not be well-suited for fluorine-lined pores such as those of our nCOF. Uptake of CO 2 at 195 K is ~270 cm 3 g −1 , a value among the highest observed for noncovalently connected structures. On the other hand, even at 90% relative humidity, crystals of 1 take up a negligible amount of H 2 O vapour ( Supplementary Fig. 7 ), consistent with their highly hydrophobic character. Hydrophobic behaviour was also confirmed by contact angle measurements with H 2 O, which revealed a contact angle of 132±1°. While this hydrophobicity has little precedent among the porous molecular crystals, fluorinated organic ligands were employed by Omary et al. [36] , [37] , [38] in the construction of very hydrophobic fluorinated MOFs, which were in turn used for hydrocarbon capture. We have subsequently expanded on this work by developing routes to larger perfluorinated ligands [39] , while Nguyen and Cohen [40] used postsynthetic functionalization of amine-bearing MOFs with long-chain acyl chlorides to create superhydrophobic MOFs. 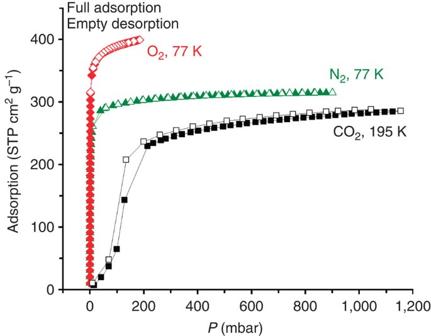Figure 4: Gas sorption in crystals of compound 1. Crystals of compound1take up N2, O2and CO2, but not H2O vapour—even at 90% relative humidity. Figure 4: Gas sorption in crystals of compound 1. Crystals of compound 1 take up N 2 , O 2 and CO 2 , but not H 2 O vapour—even at 90% relative humidity. Full size image Adsorption of liquid guests within the pores of 1 was followed by TGA [41] . We have focused on fluorocarbons, hydrocarbons [42] and CFCs [43] , [44] , [45] as guests. The experimental design is illustrated in Fig. 5 and Supplementary Fig. 8 on the example of perfluorohexane (C 6 F 14 ). Crystals of 1 were placed into the thermogravimetric balance and then heated to 120 °C, at which temperature they were kept for 1 h. The objective of this step was to remove any residual solvent and/or volatile guests from the pores of 1 . The heating was then discontinued and the material was allowed to cool down to room temperature. At that point, the flow of carrier gas was switched from pure nitrogen to nitrogen that was allowed to pass over a reservoir containing the liquid guest of interest. Using this methodology, we determined uptake capacities for several hydrocarbon and halogenated hydrocarbon guests shown in Table 1 (see also Supplementary Figs 9–15 ). Reversibility of this process was confirmed by performing over 20 adsorption/desorption cycles with perfluorohexane as the guest (see Supplementary Fig. 8 ); no loss of capacity was observed. In the case of fluorinated guests, the uptake is very fast: compound 1 gets saturated with perfluorohexane in less than 20 s (see Supplementary Fig. 8 ). At room temperature, all of the examined guests can be removed completely and within minutes from the pores of 1 if vacuum is applied. However, if vacuum is not applied, fluorinated guests will remain in the pores of 1 even after the flow of guest-enriched nitrogen is stopped; this behaviour, along with the very fast uptake, suggests high fluorophilicity of 1 . The last three guests in Table 1 are of particular interest because of their high greenhouse potential, which is hundreds to thousands of times more severe than that of CO 2 [46] . The high weight sorption percentages profit from the absence of metals in the lightweight structure of 1 . 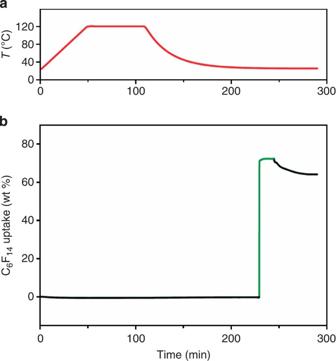Figure 5: Sorption of perfluorohexane in crystals of 1. Crystals of1take up close to 75% of their own weight in perfluorohexane. (a) The temperature program used. (b) Uptake of the guest as the function of time. Inbthe black lines indicate the parts of the program when1was exposed only to nitrogen stream, while the green line describes the section of the program when nitrogen carrying C6F14vapours was passed over1. Note that the guest remains in pores of1even after the flow of C6F14-enriched nitrogen is switched off. Figure 5: Sorption of perfluorohexane in crystals of 1. Crystals of 1 take up close to 75% of their own weight in perfluorohexane. ( a ) The temperature program used. ( b ) Uptake of the guest as the function of time. In b the black lines indicate the parts of the program when 1 was exposed only to nitrogen stream, while the green line describes the section of the program when nitrogen carrying C 6 F 14 vapours was passed over 1 . Note that the guest remains in pores of 1 even after the flow of C 6 F 14 -enriched nitrogen is switched off. Full size image Table 1 Sorption capacities and other characteristics of guest adsorbed within the pores of compound 1. Full size table In conclusion, we have synthesized and exhaustively characterized extensively fluorinated trispyrazole 1 , which assembles into a porous organic structure held together through an unusual, but highly robust combination of hydrogen bonding and [π···π] stacking. This material is lightweight, thermally and hydrolytically stable and is a superb adsorbent for hydrocarbons and their halogenated derivatives, many of which are potent greenhouse gases. This study opens up several questions [42] . Can the arms of 1 be extended to yield an isoreticular series [47] of more porous structures? Can pyrazole be replaced with other functionalities that could allow the dissection and fine tuning of hydrogen bonding and [π···π] stacking effects? Can the structure of 1 be postsynthetically [48] , [49] (or even presynthetically?) modified through nucleophilic aromatic substitutions of fluorines attached to the aromatic rings with other nucleophiles? Our current work explores these questions, and its results will be reported in due course. General methods and materials Schlenk flasks or vials with PTFE/Liner caps were used as reaction vessels for the synthesis of precursors, while standard scintillation bottles were used as vessels for the synthesis of compound 1 >. Solvents THF, Et 2 O and pentane were dried over activated alumina in an mBraun solvent purification system. Flash chromatography was performed on 60 Å silica gel (Sorbent Technologies). Gas chromatography–mass spectrometry analyses were performed on a Shimadzu GCMS-QP5000 chromatograph equipped with a Restek column (Rtx-XLB, 30 m × 0.25 mm internal diameter). The 1 H and 19 F NMR spectra were recorded on JEOL ECA-500 or ECX-400P spectrometers using the peaks of tetramethylsilane or residual solvent as standards. Trifluorotoluene (PhCF 3 , δ =−63.72 p.p.m.) was used as the internal standard in 19 F NMR spectra. 13 C Spectra were not included since they are not informative, due to poor solubility of the prepared compounds and extensive coupling between 13 C and 19 F nuclei, low intensities and many missing peaks were observed. Melting points were measured in a Barnstead International Mel-TEMP apparatus, and are uncorrected. Analytical thin-layer chromatography was performed on Fluka silica gel/TLC plates with a fluorescent indicator that emitted when irradiated at 254 nm. Infrared spectra were recorded on a Perkin-Elmer Spectrum 100 FT-IR spectrophotometer using Pike MIRacle Micrometer pressure clamp. Microanalyses were conducted by Intertek USA Inc. TGA were carried out on a TA Instruments TGA 2050 thermogravimetric analyzer at a temperature ramping rate of 2 °C min −1 under the flow of N 2 or air. DSC measurement was performed on a Mettler Toledo gas controller DSC system. Crystalline sample was placed in an aluminium crucible, heated up to 300 °C and then cooled down to −150 °C at a rate of 20 °C min −1 under N 2 . The following starting materials and solvents were obtained from the respective commercial sources and used without further purification: Boc 2 O (Alfa Aesar); triphenylchloromethane (TrCl) (AK Scientific); N , N -dimethylformamide (DMF), and NaN 3 (TCI America); Perfluorohexane, 1,1,2-trichlorotrifluoroethane (CFC-113) and 3,3-dichloro-1,1,1,2,2-pentafluoropropane (HCFC-225ca) (SynQuest Labs); lithium t-butoxide (t-BuOLi) (Strem); 2,3,5,6-tetrafluorobenzene, triethylamine (Et 3 N), tetrakis(triphenylphosphine)palladium(0) (Pd(PPh 3 ) 4 ), 4-iodopyrazole and trifluoroacetic acid (TFA) (Matrix Scientific); methanol, toluene, n -hexane, dichloromethane, chloroform, cyclohexane (Aldrich); water (Milli-Q, deionized). All gases were purchased from Matheson Tri-Gas. Synthesis of compound 4 A 500-ml screw cap pressure vessel was equipped with magnetic stir bar and charged with CuCl (15.0 g, 150 mmol) and t -BuOLi (12.0 g, 150 mmol). Dry DMF (240 ml) was added. The reaction vessel was sealed, taken out of the glovebox, sonicated for 5 min and then vigorously stirred at 25 °C for 1 h. The pressure vessel was placed back inside the glovebox. Tetrafluorobenzene (52.5 g, 350 mmol) was added in one portion, the reaction vessel was sealed, taken out of the glovebox, sonicated for 5 min and vigorously stirred at 25 °C for 1 h. The pressure vessel was placed back inside the glovebox. Catalyst Pd(PPh 3 ) 4 (1.15 g, 1.00 mmol) was added, followed by N -trityl-4-iodopyrazole [50] ( 3 , 43.6 g, 100 mmol). Reaction mixture was sealed, taken out of the glovebox and then placed inside an oil bath preheated to 100 °C, where it was stirred vigorously for 12 h. Reaction mixture was cooled to 25 °C, diluted with CH 2 Cl 2 (500 ml) and 3% aqueous citric acid (400 ml) was added. Reaction mixture was filtered through the plug of Celite to remove CuI. Filter cake was washed with additional CH 2 Cl 2 (3 × 50 ml). Combined organic layers were separated and washed with deionized water (5 × 350 ml), followed by brine (250 ml). Finally, the organic layer was dried over anhydrous MgSO 4 , filtered and dry-absorbed on silica gel. After purification by column chromatography on silica gel using CH 2 Cl 2 /hexanes (gradient from 50 to 90% of CH 2 Cl 2 ) as eluent and evaporation of the fractions containing the product, title compound was obtained as a tan oil (39.0 g, 85%). R f =0.46 (SiO 2 , hexanes/CH 2 Cl 2 1/1). 1 H NMR (400 MHz, CDCl 3 , Supplementary Fig. 16 ): δ 8.21 (s, 1H), 7.98 (s, 1H), 7.40–7.30 (m, 9H), 7.22–7.15 (m, 6H), 6.96–6.84 (m, 1H) p.p.m. 19 F NMR (376 MHz, CDCl 3 , Supplementary Fig. 17 ): δ −139.7 to −139.8 (m, 2F), −141.1 to −141.3 (m, 2F) p.p.m. High-resolution mass spectrum (HRMS) (CI + mode): calculated for C 28 H 18 F 4 N 2 458.1406. found: 458.1401. Synthesis of compound 5 A 100-ml screw cap pressure vessel was equipped with a magnetic stir bar and charged with CuCl (3.35 g, 33.5 mmol) and t -BuOLi (2.68 g, 33.5 mmol). Dry DMF (40 ml) was added, and the vessel was sealed, taken out of the glovebox, sonicated for 5 min and vigorously stirred at 25 °C for 1 h. The pressure vessel was then placed back inside the glovebox, and compound 4 (15.6 g, 34.0 mmol) was added in one portion. After that, the reaction vessel was sealed again, taken out of the glovebox, sonicated for 5 min and vigorously stirred at 25 °C for 1 h. The pressure vessel was placed back inside the glovebox. Catalyst Pd(PPh 3 ) 4 (347 mg, 0.30 mmol) was added, followed by 1,3,5-triiodobenzene (4.56 g, 10 mmol). The reaction vessel was sealed, taken out of the glovebox and placed inside an oil bath preheated to 100 °C, where it was stirred vigorously for 12 h. Reaction mixture was cooled to 25 °C, diluted with CH 2 Cl 2 (150 ml) and 3% aqueous citric acid (100 ml) was added. After filtration through a plug of Celite, the filter cake was washed with additional CH 2 Cl 2 (3 × 25 ml). Combined organic layers were separated and washed with deionized water (5 × 100 ml), followed by brine (100 ml). The organic layer was dried over anhydrous MgSO 4 , filtered and dry-absorbed on silica gel. After purification by column chromatography on silica gel using CH 2 Cl 2 /hexanes as eluent and evaporation of the fractions containing the product, compound 5 was obtained as a tan oil (13.5 g, 93%). R f =0.74 (SiO 2 , CH 2 Cl 2 ). 1 H NMR (400 MHz, CDCl 3 , Supplementary Fig. 18 ) δ 8.20 (s, 1H), 7.96 (s, 1H), 7.67 (s, 1H) 7.40–7.30 (m, 27H), 7.22–7.15 (m, 18H) p.p.m. 19 F NMR (376 MHz, CDCl 3 , Supplementary Fig. 19 ) δ −140.6 to −140.8 (m, 6F), −144.6 to −144.9 (m, 6F) p.p.m. This compound was used as crude in the next step. Synthesis of compound 6 A 250-ml flask equipped with a magnetic stir bar was charged with compound 5 (13.3 g, 9.20 mmol) and CHCl 3 (140 ml). The resulting clear solution was stirred vigorously and then trifluoroacetic acid (12 ml) was added, resulting in a colour change from colourless to yellow. Stirring was continued at 25 °C for 20 h. Resulting salt that was formed during the reaction was filtered off and washed with fresh CHCl 3 (3 × 50 ml). Obtained light tan solid was dried in vacuum for 2 h. A 250-ml flask equipped with a magnetic stir bar was charged with this isolated salt and CH 2 Cl 2 (100 ml) was added. The resulting suspension was treated with Et 3 N (9 ml), followed by the addition of 4-dimethylaminopyridine (1.22 g, 10.0 mmol). To the open flask Boc 2 O (12.0 g, 55 mmol) was added via a syringe over 5 min. CAUTION: rapid evolution of CO 2 is observed during the addition! After addition of Boc 2 O was complete, the reaction flask was capped with a septum connected to a bubbler. Reaction mixture was stirred vigorously at 25 °C until the evolution of CO 2 ceased (typically 12–36 h). Upon completion, the reaction mixture was dry-absorbed on silica gel. After purification by column chromatography on silica gel (using EtOAc/CH 2 Cl 2 as eluent) and evaporation of the fractions containing the product, compound 6 was obtained as a white solid (5.3 g, 56% over two steps), mp 350 °C (decomposition). 1 H NMR (500 MHz, CDCl 3 , Supplementary Fig. 20 ) δ 8.65 (s, 3H), 8.25 (s, 3H), 7.78 (s, 3H), 1.71 (s, 27 H) p.p.m. 19 F NMR (470 MHz, CDCl 3 , Supplementary Fig. 21 ) δ −139.8 to −140.0 (m, 6F), −143.7 to −143.9 (m, 6F) p.p.m. Fourier transform infrared spectroscopy (FT-IR) ( Supplementary Fig. 22 ): 3,213 (s, N=C–H ), 3,140 (s, N–C–H ), 2,985 (m, C=C–H ), 1,794 (m, C=O ), 1,759 (m, C=N ), 1,581 (s, C=C ), 1,498 (s), 1,481 (s), 1,400 (s), 1,375 (s), 1,348 (s), 1,296 (s), 1,246 (s), 1,153 (s), 1,033 (m), 972 (s), 845 (s) cm −1 . HRMS (ESI + mode): calculated for C 48 H 36 F 12 N 6 O 6 Na: 1,043.23970. Found: 1,043.23810. Synthesis and stability testing of compound 1 Compound 6 (200 mg, 0.20 mmol) was added to a 100-ml glass bottle. Solvents DMF (20 ml) and MeOH (20 ml) were added to the solid and the mixture was sonicated for 10 min. The bottle was capped and placed into an 80 °C oven for 1 day. The resulting colourless rod-shape crystals (mp >350 °C) were washed with MeOH and air-dried. The yield of 1 was 92%, calculated from the dried sample. 1 H NMR (500 MHz, DMSO- d 6 , Supplementary Fig. 23 ) δ 13.54 (s, 3H), 8.36 (s, 3H), 8.03 (s, 3H), 7.95 (s, 3H) p.p.m. 19 F NMR (470 MHz, DMSO- d 6 , Supplementary Fig. 24 ) δ −141.5 to −141.6 (m, 6F), −144.7 to −144.9 (m, 6F) p.p.m. FT-IR ( Supplementary Fig. 25 ): 3,469 (m, N–H ), 3,213 (s, N=C–H ), 3,147 (s, N–C–H ), 2,966 (m, C=C–H ), 1,653 (m, C=N ), 1,570 (s, C=C ), 1,491 (s), 1,427 (s), 1,394 (s), 1,342 (m), 1,219 (m), 1,155 (m), 1,025 (s), 980 (s), 962 (s), 949 (m), 804 (s) cm −1 . Anal. calcd (%) for C 33 F 12 H 12 N 6 : C 54.99, H 1.68, N 11.66; found: C 54.61, H 1.46, N 11.56. HRMS (CI + mode): calculated for C 33 H 12 F 12 N 6 : 720.0932. Found: 720.0926. Compound 1 could be sublimed using the following procedure. A 30-cm-long quartz tube containing a sample of compound 1 was connected to a vacuum source (0.03 mm Hg) and the bottom half of the tube was heated in a 250 °C oven with 1 °C min −1 heating rate. White microcrystalline solid was collected from the wall of the cold part of the tube above the oven after 48 h. The solid was ground in a mortar and its PXRD pattern was compared with the sample obtained by solvothermal synthesis (see Supplementary Fig. 5 ). Stability of compound 1 to various solvents was tested by exposing a handful of crystals to the given solvent and observing them visually over time. If—under given conditions—no visible signs of crystal decomposition of dissolution were observed, the crystals were harvested and subjected to PXRD analysis ( Supplementary Fig. 1 ). If PXRD patterns also appeared unchanged, compound 1 was deemed stable to those conditions. Using this methodology, we have determined 1 to be stable to: deionized H 2 O at 25 °C for at least 30 days, and at 100 °C for at least 7 days; 2 M aqueous solution of NaOH and 1 M aqueous solution of HCl at 25 °C for at least 30 days; CH 2 Cl 2 at 25 °C for at least 30 days; hexanes at 25 °C for at least 30 days; acetone at 25 °C for at least 30 days; and toluene at 25 °C for at least 30 days. Compound 1 is sparingly soluble in DMSO at 25 °C, but its solubility in this solvent considerably increases with temperature. PXRD patterns of compound 1 The synchrotron PXRD data of compound 1 were collected at the BL01C2 beamline at the National Synchrotron Radiation Research Center in Taiwan. The wavelength of the incident X-rays was 1.03321 Å and the diffraction patterns were recorded with a Mar345 IP detector, positioned ~306 mm from the sample. The powder sample was packed in a glass capillary (0.3 mm diameter) and each pattern was exposed for 60 s. In situ temperature-dependent diffraction data on compound 1 were collected in a stream of hot air at temperatures of 25, 100, 150, 200, 250, 300 and 350 °C, with a heating rate of 10 °C min −1 . Every set point of the temperature gradient was sustained for 10 min to ensure the temperature balance in the entire powder sample. The one-dimensional powder diffraction profile was converted using GSAS-II package [51] with cake-type integration, where the diffraction angles were calibrated according to Bragg positions of LaB 6 standard from National Institute of Standards and Technology (NIST). Simulated PXRD patterns were calculated with the Material Studio software package [52] employing the structure model from the obtained single-crystal data. PXRD data of sublimed compound 1 were collected at 25 °C on a Phillips X'pert Pro diffractometer with CuKα radiation. Gas adsorption A Micromeritics ASAP 2020 Surface Area and Porosity Analyzer was used to measure N 2 , O 2 , CO 2 and H 2 O adsorption isotherms. Oven-dried sample tubes equipped with seal frit (Micrometrics) were evacuated and tared. Samples of 1 weighing between 100 and 200 mg were transferred to the sample tube, which was then capped by a seal frit. Samples were heated to 120 °C under high vacuum (10 −3 –10 −4 Torr) for 15 h. The evacuated sample tubes were weighed again, and the sample mass was determined by subtracting the mass of the previously tared tubes. Isotherms for the sorption of N 2 and O 2 were measured using a liquid nitrogen bath (77 K). Isotherm for the sorption of CO 2 was measured using a dry ice/isopropanol bath (195 K). Water vapour adsorption isotherm was measured at 298 K using a water bath. Ultra high purity grade (99.999%) gases—N 2 , O 2 , CO 2 and He—as well as oil-free valves and gas regulators were used for all free-space corrections and measurements. Relative pressure ( P / P 0 ) range for Brunauer–Emmett–Teller analysis was taken from 5 × 10 −5 to 0.1. Contact angle measurements Finely ground crystals of compound 1 were pressed between two Si(100) slides that had been previously rinsed with absolute EtOH and dried in a stream of N 2 gas. After removing the upper slide, the exposed crystal surface was used for conducting contact angle measurements. A ramé-hart model 100 contact angle goniometer was employed to measure the contact angle of H 2 O and compound 1 . The contacting liquid was dispensed on the surface of the compound 1 using a Matrix Technologies micro-Electrapette 25 at the slowest speed of 1 μl s −1 . The measurements were performed at 293 K, with the pipet tip remaining in contact with the drop. The reported data for each sample were the average of three measurements obtained from three different slides for compound 1 with advancing contact angles ( θ a ) recorded for both edges of the drop. Thermogravimetric vapour adsorption Colourless rod crystals of compound 1 were first heated on a thermobalance of the TA Instruments TGA 2050 thermogravimetric analyzer under N 2 flow to 120 °C. They were then held at this temperature for 60 min to ensure complete activation. After no further weight change could be noticed, the temperature was reduced to 25 °C at 5 °C min −1 and held at 25 °C. The N 2 flow was then switched (green line) to a second N 2 gas stream that was saturated with the vapour of adsorbate at 25 °C (saturation was achieved by passing the N 2 gas stream through a bubbler containing the liquid adsorbate). After the weight reached a plateau, the adsorbate vapour/N 2 flow was switched back to pure N 2 flow at the same temperature (25 °C). Accession codes: The X-ray crystallographic coordinates for structures reported in this Article have been deposited at the Cambridge Crystallographic Data Centre (CCDC), under deposition number CCDC 1004205. These data can be obtained free of charge from The Cambridge Crystallographic Data Centre via www.ccdc.cam.ac.uk/data_request/cif . How to cite this article: Chen, T.-H. et al. Thermally robust and porous noncovalent organic framework with high affinity for fluorocarbons and CFCs. Nat. Commun. 5:5131 doi: 10.1038/ncomms6131 (2014).